Cidea improves the metabolic profile through expansion of adipose tissue In humans, Cidea (cell death-inducing DNA fragmentation factor alpha-like effector A) is highly but variably expressed in white fat, and expression correlates with metabolic health. Here we generate transgenic mice expressing human Cidea in adipose tissues (aP2-hCidea mice) and show that Cidea is mechanistically associated with a robust increase in adipose tissue expandability. Under humanized conditions (thermoneutrality, mature age and prolonged exposure to high-fat diet), aP2-hCidea mice develop a much more pronounced obesity than their wild-type littermates. Remarkably, the malfunctioning of visceral fat normally caused by massive obesity is fully overcome—perilipin 1 and Akt expression are preserved, tissue degradation is prevented, macrophage accumulation is decreased and adiponectin expression remains high. Importantly, the aP2-hCidea mice display enhanced insulin sensitivity. Our data establish a functional role for Cidea and suggest that, in humans, the association between Cidea levels in white fat and metabolic health is not only correlative but also causative. Cidea (cell death-inducing DNA fragmentation factor alpha-like effector A) is a lipid droplet-associated protein [1] , [2] . In humans, Cidea is highly but variably expressed in white fat [3] , [4] . A low expression level of Cidea in human fat is associated with several features of the metabolic syndrome [3] . Conversely, Cidea expression is high in adipose tissues of obese subjects with preserved insulin sensitivity [1] . Furthermore, changes in adipose tissue Cidea mRNA levels parallel variations in insulin sensitivity independently of changes in body mass index [5] . Thus, in humans, Cidea is positively correlated with insulin sensitivity and healthy obesity. However, it is unknown whether Cidea actually causes the metabolically healthy phenotype or merely reflects the better metabolic state. In mice, Cidea is not expressed in white adipose tissue but is highly expressed in brown and brite adipocytes [6] , [7] , [8] . Therefore, mouse models open opportunities to establish a possible causative effect of Cidea in conferring health to an obese phenotype. Using this opportunity, we humanized mice by introducing human Cidea into their white fat. We further performed all metabolic examinations under conditions approaching human conditions—at thermoneutral temperature (where the thermal drive for heat production to combat heat loss is eliminated [9] ), in mature mice (when the experiments were initiated, the mice were 12-week old, that is, fully developed) and with exposure of the mice to a westernized diet (high-fat diet) for 6–8 months, that is, a time sufficiently long to reflect the chronic human conditions under which an obese or lean phenotype develops and mimicking the relative age of obese humans. We demonstrate that, under these humanized conditions, aP2-hCidea mice gained much more weight than wild-type mice. Despite being significantly more obese, aP2-hCidea mice displayed ameliorated insulin sensitivity. Thus, the transgenic mice developed a metabolically healthy obesity, pointing to Cidea as being an important and causative factor involved in protection against the metabolic complications of obesity. Generation and characterization of aP2-hCidea mice To create transgenic mice expressing human Cidea in white fat, we utilized a full-length aP2 promoter/enhancer, which is adipose tissue-selective and active during fat cell differentiation ( Fig. 1a ) [10] , [11] . We developed several founder lines of aP2-hCidea mice ( Fig. 1b,c and Supplementary Fig. 1 ). The line (line 13), in which human Cidea protein in white adipose tissues (WAT) (gonadal (gWAT) and inguinal (iWAT)) was expressed at physiological levels (similar to the endogenous Cidea levels in interscapular brown fat; Fig. 1b ), was used to examine the phenotype further. The human Cidea protein expressed in vivo had a similar size to human Cidea protein produced in vitro ( Fig. 1c ). Quantitative reverse transcription–PCR for the human Cidea confirmed that expression was largely confined to adipose tissues with little or no expression in other tissues ( Fig. 1d , right panel). Endogenous Cidea under standard temperature conditions was almost exclusively expressed in brown fat ( Fig. 1d , left panel). The phenotype described here is therefore due primarily to expression of Cidea in adipose tissues. 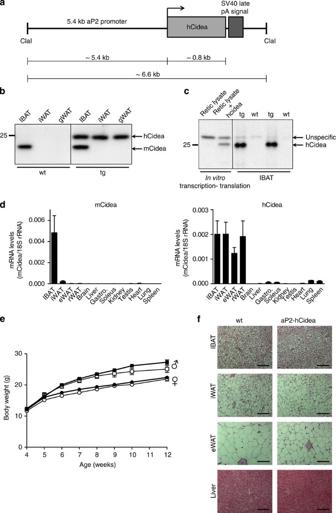Figure 1: Generation of aP2-hCidea transgenic mice. (a) Schematic diagram of the transgenic construct; an aP2 enhancer/promoter (from −5.4 kb to +21 bp) was fused to the human Cidea (hCidea) coding sequence followed by the SV40 late polyadenylation signal. (b–d) Tissue-specific expression of human and mouse Cidea in aP2-hCidea transgenic mice. (b) Protein levels of human Cidea and mouse Cidea (mCidea) in adipose tissues. Western blot, performed with an antibody recognizing both human and mouse Cidea, demonstrates the presence of human Cidea protein in both brown and white adipose tissues (inguinal (iWAT) and gonadal (gWAT)) of transgenic mice; mouse Cidea protein is expressed only in interscapular brown adipose tissue (IBAT) in both transgenic and wild-type mice. (c) Expression of human Cidea protein in IBAT of transgenic mice. Western blot, performed with a human-only Cidea-specific antibody, demonstrates the presence of human Cidea protein only in transgenic mice (right part); its size is similar to the size of human Cidea protein generatedin vitro(left part). (d) mRNA levels of mouse Cidea (mCidea; left panel) and human Cidea (hCidea; right panel) in adipose tissues and multiple organs. Data are means±s.e.m. from three transgenic mice. (e) Body weights of wild-type mice (open symbols; males, open squares,n=8; females, open circles,n=4) and aP2-hCidea mice (filled symbols; males, filled squares,n=14; females, filled circles,n=10) from weaning (4 weeks of age) until 12 weeks of age, at room temperature and on chow diet. (f) Histological appearance of IBAT, iWAT, eWAT and liver of 12-week-old wild-type and aP2-hCidea mice (as ine). Paraffin sections (5 μm thick) were stained with haematoxylin and eosin. Scale bar, 100 μm. Figure 1: Generation of aP2-hCidea transgenic mice. ( a ) Schematic diagram of the transgenic construct; an aP2 enhancer/promoter (from −5.4 kb to +21 bp) was fused to the human Cidea (hCidea) coding sequence followed by the SV40 late polyadenylation signal. ( b – d ) Tissue-specific expression of human and mouse Cidea in aP2-hCidea transgenic mice. ( b ) Protein levels of human Cidea and mouse Cidea (mCidea) in adipose tissues. Western blot, performed with an antibody recognizing both human and mouse Cidea, demonstrates the presence of human Cidea protein in both brown and white adipose tissues (inguinal (iWAT) and gonadal (gWAT)) of transgenic mice; mouse Cidea protein is expressed only in interscapular brown adipose tissue (IBAT) in both transgenic and wild-type mice. ( c ) Expression of human Cidea protein in IBAT of transgenic mice. Western blot, performed with a human-only Cidea-specific antibody, demonstrates the presence of human Cidea protein only in transgenic mice (right part); its size is similar to the size of human Cidea protein generated in vitro (left part). ( d ) mRNA levels of mouse Cidea (mCidea; left panel) and human Cidea (hCidea; right panel) in adipose tissues and multiple organs. Data are means±s.e.m. from three transgenic mice. ( e ) Body weights of wild-type mice (open symbols; males, open squares, n =8; females, open circles, n =4) and aP2-hCidea mice (filled symbols; males, filled squares, n =14; females, filled circles, n =10) from weaning (4 weeks of age) until 12 weeks of age, at room temperature and on chow diet. ( f ) Histological appearance of IBAT, iWAT, eWAT and liver of 12-week-old wild-type and aP2-hCidea mice (as in e ). Paraffin sections (5 μm thick) were stained with haematoxylin and eosin. Scale bar, 100 μm. Full size image General phenotype Transgenic aP2-hCidea mice were born at the expected frequency, with no observed signs of abnormality, illness or increased mortality at least up to 1 year of age. On chow diet at room temperature, aP2-hCidea and wild-type mice gained weight to a similar extent ( Fig. 1e ). No anatomic abnormalities were observed on gross or light microscopic examination of 12-week-old mice ( Fig. 1f ). Under humanized conditions aP2-hCidea mice are more obese To mimic the human situation, wild-type mice and the transgenic mice were fed an obesogenic (high-fat) diet at thermoneutrality for a prolonged time (6–8 months). The expression of hCidea in white fat had remarkable effects on the energy metabolism of the mice. They gained substantially more body weight than their wild-type littermates. This was entirely due to an increase in fat mass ( Fig. 2a–c ); there was no effect on lean mass ( Supplementary Fig. 2b ). In mice undisturbed by frequent examination, the difference in obesity was manifested much earlier ( Supplementary Fig. 2c ). The increase in body and fat weight in the transgenic mice could not be readily explained by a significant increase in food intake ( Fig. 2d ) or a significant decrease in daily energy expenditure ((EE); Supplementary Fig. 3 ) [12] , although both measures tended to deviate in the energy accumulative direction. Metabolic efficiency, that is, the percentage of consumed energy incorporated into fat, was substantially higher in the aP2-hCidea mice ( Fig. 2d–f ). 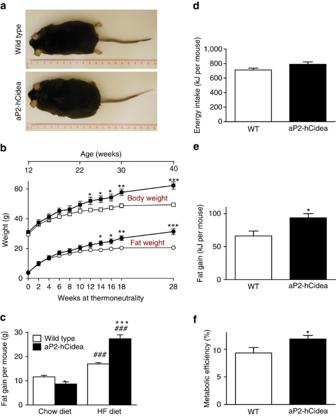Figure 2: aP2-hCidea mice become more obese. (a) Appearance of wild-type and transgenic mice after 34 weeks on high-fat diet at thermoneutrality. (b) Body composition of wild-type (open symbols) (n=7) and transgenic mice (filled symbols;n=6) during 28 weeks on high-fat diet. The mice were 12-week-old when the experiment started. (c) Average fat gain after 28 weeks at thermoneutrality on chow or high-fat diet; based onbandSupplementary Fig. 2a. (d–f) Total energy intake (d) and total fat gain (e) of wild-type (n=10) and transgenic mice (n=11) between weeks 8 and 10 on high-fat diet. (f) Metabolic efficiency. Values represent percentage of consumed energy incorporated into fat (calculated as (fat weight gained (kJ)/energy intake (kJ)) × 100); based ond,e. Values shown in all panels are means±s.e.m. *Significant difference between genotypes; *P<0.05; **P<0.01; ***P<0.001 by Student’st-test.#Significant difference between diets;###P<0.001 by Student’st-test. Figure 2: aP2-hCidea mice become more obese. ( a ) Appearance of wild-type and transgenic mice after 34 weeks on high-fat diet at thermoneutrality. ( b ) Body composition of wild-type (open symbols) ( n =7) and transgenic mice (filled symbols; n =6) during 28 weeks on high-fat diet. The mice were 12-week-old when the experiment started. ( c ) Average fat gain after 28 weeks at thermoneutrality on chow or high-fat diet; based on b and Supplementary Fig. 2a . ( d – f ) Total energy intake ( d ) and total fat gain ( e ) of wild-type ( n =10) and transgenic mice ( n =11) between weeks 8 and 10 on high-fat diet. ( f ) Metabolic efficiency. Values represent percentage of consumed energy incorporated into fat (calculated as (fat weight gained (kJ)/energy intake (kJ)) × 100); based on d , e . Values shown in all panels are means±s.e.m. *Significant difference between genotypes; * P <0.05; ** P <0.01; *** P <0.001 by Student’s t -test. # Significant difference between diets; ### P <0.001 by Student’s t -test. Full size image On high-fat diet Cidea promotes adipose tissue expansion In animals on chow diet, inguinal (iWAT) and epididymal (eWAT) adipose tissues were somewhat smaller in the transgenic mice ( Fig. 3a , left-hand red cross in each panel, in agreement with Supplementary Fig. 2a ). 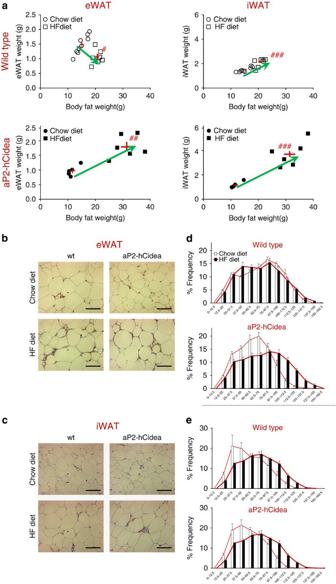Figure 3: Cidea promotes adipose tissue expansion. (a) Weight of white adipose tissues (epididymal (eWAT) and inguinal (iWAT)) expressed as a function of body fat weight. Wild-type and transgenic mice had been on chow (wt,n=8–9; tg,n=5) or high-fat diet (wt,n=7; tg,n=6) at thermoneutrality for 28 weeks. Crosses represent mean values±s.e.m. Arrows denote the direction of adipose tissue weight changes induced by high-fat diet.#Significant difference between diets;#P<0.05;##P<0.01;###P<0.001 by Student’st-test. (b–c) Histological appearance of eWAT (b) and iWAT (c; mice on diets for 34 weeks). Paraffin sections (5 μm thick) were stained with haematoxylin and eosin. Scale bar, 100 μm. (d–e) Analysis of adipocyte size distribution in eWAT (d) and iWAT (e) of wild-type and transgenic mice on chow or high-fat diet. Values are mean frequencies of cell diameter±s.e.m. calculated from a minimum of 500 cells per animal with 4–7 animals per group. Figure 3: Cidea promotes adipose tissue expansion. ( a ) Weight of white adipose tissues (epididymal (eWAT) and inguinal (iWAT)) expressed as a function of body fat weight. Wild-type and transgenic mice had been on chow (wt, n =8–9; tg, n =5) or high-fat diet (wt, n =7; tg, n =6) at thermoneutrality for 28 weeks. Crosses represent mean values±s.e.m. Arrows denote the direction of adipose tissue weight changes induced by high-fat diet. # Significant difference between diets; # P <0.05; ## P <0.01; ### P <0.001 by Student’s t -test. ( b – c ) Histological appearance of eWAT ( b ) and iWAT ( c ; mice on diets for 34 weeks). Paraffin sections (5 μm thick) were stained with haematoxylin and eosin. Scale bar, 100 μm. ( d – e ) Analysis of adipocyte size distribution in eWAT ( d ) and iWAT ( e ) of wild-type and transgenic mice on chow or high-fat diet. Values are mean frequencies of cell diameter±s.e.m. calculated from a minimum of 500 cells per animal with 4–7 animals per group. Full size image Although all mice on high-fat diet became obese (compare Fig. 2b and Supplementary Fig. 2a ), it is remarkable that in wild-type mice, only iWAT had expanded ( Fig. 3a , top-right panel), whereas the weight of eWAT was actually decreased ( Fig. 3a , top-left panel; principally in accordance with refs 13 , 14 ). In transgenic mice, high-fat diet led to much more dramatic iWAT expansion (its average weight was increased more than three times; Fig. 3a , bottom-right panel). However, the decrease of eWAT seen in wild-type mice was not only abolished in transgenic mice, but also the tissue was even further expanded ( Fig. 3a , bottom-left panel). Thus, the qualitatively different consequences of Cidea presence were observed only in eWAT. It is noteworthy that the subcutaneous (iWAT) and the visceral (eWAT) adipose depots are known to respond differently to prolonged exposure to a high-fat diet. Hyperplasia is initiated in eWAT but not in iWAT [15] , [16] , and eWAT is highly susceptible to obesity-associated adipocyte death, whereas iWAT is relatively resistant [13] . Thus, both the plasticity and the expandability of eWAT were rescued by the presence of Cidea. Correspondingly, fat deposition in the liver was lower in aP2-hCidea mice (20±1% versus 23±2% in wild-type mice, P <0.05 by Student’s t -test). There was no effect on blood triglyceride and glycerol levels ( Supplementary Table 1 ). In eWAT of the transgenic mice on chow diet, the adipocytes were smaller than in wild-type mice ( Fig. 3b , left panels, Supplementary Fig. 4a and Supplementary Table 2 ). They were also smaller than the adipocytes of the transgenic mice on high-fat diet ( Fig. 3b , bottom panels, Fig. 3d and Supplementary Table 2 ). Thus, a high-fat diet-induced expansion of eWAT in transgenic mice could, at least in part, be explained by adipocyte hypertrophy. Remarkably, these adipocytes had perfectly spherical shape ( Fig. 3b , bottom-right panel). In contrast, adipocytes of wild-type mice on high-fat diet had irregular polygonal shape, a feature of stressed adipose cells [17] ( Fig. 3b , top-right panel). The average diameter of iWAT adipocytes was similar in wild-type and transgenic mice on either of diets ( Fig. 3c , Supplementary Fig. 4c,d and Supplementary Table 2 ). High-fat diet led to similar increases in iWAT adipocyte diameter in both genotypes ( Fig. 3e and Supplementary Table 2 ). Macrophage infiltration not determinative High-fat diet led to an increase in total protein content in both adipose depots, in both genotypes ( Fig. 4a ). However, high-fat diet led to an increase in protein density (that is, protein levels normalized to tissue weight) only in eWAT of wild-type mice ( Fig. 4b ), highlighting significant differences in tissue composition between wild-type and transgenic mice. Histological analysis of eWAT of wild-type mice indicated that the increased protein density could not be explained by reduced adipocyte size ( Fig. 3b,d and Supplementary Table 2 ); the size of adipocytes in wild-type mice on chow and on high-fat diet appeared to be similar. By visual inspection, it was observed that high-fat feeding led to a clearly augmented number of macrophages only in eWAT (compare Fig. 3b,c ). Thus, the increase in protein density in eWAT of wild-type mice could potentially be explained by a massive macrophage infiltration [13] , [18] , [19] , [20] , [21] . 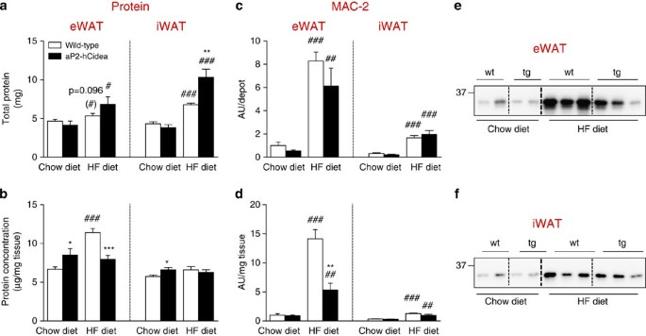Figure 4: Cidea does not prevent adipose tissue-macrophage infiltration. (a–d) Total protein content (a), protein density (b), MAC-2 protein content (c) and MAC-2 protein density (d) in eWAT and iWAT of wild-type (white bars) and transgenic mice (black bars) that have been on chow (wt,n=9; tg,n=5) or high-fat diet (wt,n=7; tg,n=6) at thermoneutrality for 28 weeks. Values are means±s.e.m. *Significant difference between genotypes; *P<0.05; **P<0.01; ***P<0.001 by Student’st-test.#Significant difference between diets;#P<0.05;##P<0.01;###P<0.001 by Student’st-test. (e–f) Representative western blots of MAC-2 in eWAT (e) and iWAT (f). Figure 4: Cidea does not prevent adipose tissue-macrophage infiltration. ( a – d ) Total protein content ( a ), protein density ( b ), MAC-2 protein content ( c ) and MAC-2 protein density ( d ) in eWAT and iWAT of wild-type (white bars) and transgenic mice (black bars) that have been on chow (wt, n =9; tg, n =5) or high-fat diet (wt, n =7; tg, n =6) at thermoneutrality for 28 weeks. Values are means±s.e.m. *Significant difference between genotypes; * P <0.05; ** P <0.01; *** P <0.001 by Student’s t -test. # Significant difference between diets; # P <0.05; ## P <0.01; ### P <0.001 by Student’s t -test. ( e – f ) Representative western blots of MAC-2 in eWAT ( e ) and iWAT ( f ). Full size image Obesity-induced macrophage infiltration into eWAT seemed to be lower in transgenic than in wild-type mice ( Fig. 3b , right panels). To quantify the degree of macrophage infiltration, we measured protein levels of the macrophage markers MAC-2 and F4/80. In agreement with the morphological data, high-fat diet led to a significant increase of MAC-2 protein content in both depots, in both genotypes ( Fig. 4c ). Also in agreement with the morphological data, the levels of MAC-2 in eWAT were remarkably higher than in iWAT, highlighting a much higher systemic inflammatory impact in eWAT. Macrophage marker protein densities in eWAT of transgenic mice on high-fat diet were lower ( Fig. 4d–f and Supplementary Fig. 5a , right panel), demonstrating that the number of macrophages per tissue weight was reduced compared with wild-type mice. However, the total systemic inflammatory impact in eWAT (defined as the total number of macrophages per fat depot ( Fig. 4c and Supplementary Fig. 5a , left panel)) was not different between wild-type and transgenic mice. The expression levels of proinflammatory (M1) and anti-inflammatory (M2) macrophage markers ( Supplementary Figs 6b–d and 7 ) suggested that the obesity-induced shift in M1/M2 ratio was not affected by the presence of Cidea either in eWAT or iWAT. The retained inflammation in eWAT would thus be in agreement with the recent suggestion that this is a requirement for visceral adipose expansion [22] . Picrosirius red staining of eWAT did not reveal any major histological differences in collagen deposition between wild-type and transgenic mice on either of the diets ( Supplementary Fig. 8a ). The expression levels of NLRP3 inflammasome-related genes [17] , [23] ( Supplementary Fig. 6e ), and some extracellular matrix-related genes [24] ( Supplementary Fig. 8b ) also suggest that neither pyroptosis nor adipose tissue fibrosis were significantly different between wild-type and transgenic mice. Therefore, the physiological basis of the retained eWAT expandability in transgenic mice is most likely related to the adipocytes themselves. Although aP2 was originally identified as an adipocyte-specific protein, it has been demonstrated that the aP2 promoter may also be active in macrophages (for example, see ref. 25 ). To examine the specificity of Cidea expression (that is, whether it is also expressed in adipose tissue macrophages), Cidea protein expression was measured in stromal vascular fractions of eWAT and iWAT of transgenic mice fed a high-fat diet. In comparison to whole adipose tissue, in the stromal-vascular fractions, Cidea was expressed at negligible levels ( Supplementary Fig. 5b ). The absence of Cidea protein expression in the stromal-vascular fraction of adipose tissues, as well as the absence of correlation between Cidea and macrophage marker expression ( Supplementary Fig. 5c ) are clear evidence of absence of its expression in adipose tissue macrophages and verification that it is almost entirely expressed in adipocytes (fully in agreement with [26] ). Thus, the phenotype observed in transgenic mice is fully the consequence of Cidea expression in adipocytes. Cidea preserves molecular identity of visceral adipose tissue Perilipin 1 is the most abundant protein on the surface of adipocyte lipid droplets, playing an important role in the regulation of basal and hormonally stimulated lipolysis. Cidea is also found on the surface of lipid droplets, co-localized with perilipin 1 (refs 1 , 2 ). In obese mice, in eWAT, perilipin 1 is lost in degenerated and nonviable adipocytes, whereas it is retained in viable adipocytes [13] , [27] , [28] . As eWAT of wild-type mice on prolonged high-fat diet demonstrated an inability to expand, we examined whether perilipin 1 levels were affected. As seen on Fig. 5a,b , high-fat diet-induced obesity led to a virtually complete loss of perilipin 1 in eWAT of wild-type mice. In contrast, perilipin 1 was fully retained in the eWAT of transgenic mice ( Fig. 5a,b ). Prolonged high-fat diet exerted a similar effect on the serine/threonine-specific protein kinase Akt, a key mediator of insulin signalling [29] . Akt protein levels were almost abolished in eWAT of wild-type mice, whereas they were unaffected in eWAT of transgenic mice ( Fig. 5a,b ). The effect of high-fat diet was protein-selective, as the protein levels of FABP4 were not affected ( Fig. 5a , lowest row). It was also eWAT depot specific, as the effects of high-fat diet on iWAT perilipin 1 and Akt levels were not significantly different between wild-type and transgenic mice ( Supplementary Fig. 9 ). Importantly, mRNA levels of perilipin family proteins and mRNA levels of Akt1/2 were not increased in eWAT (as well as in iWAT) of transgenic mice ( Supplementary Figs 10 and 11 ). Thus, Cidea protective effects were exerted at the posttranscriptional level. Preserved perilipin 1 and Akt retention in the visceral (eWAT) fat of transgenic mice point to Cidea being a molecule capable of protecting the visceral adipocytes against the detrimental effects of a high-fat diet. 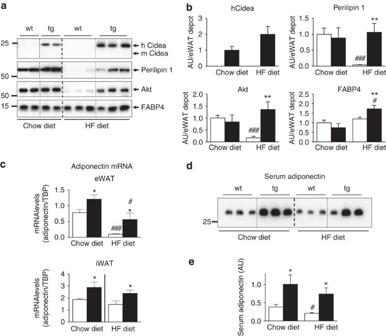Figure 5: Cidea permits perilipin retention in eWAT. (a–b) Representative western blots (a) and protein levels (b) of hCidea, perilipin 1, Akt and FABP4 in eWAT of wild-type (white bars) and transgenic mice (black bars) that have been on chow (wt,n=9; tg,n=5) or high-fat diet (wt,n=7; tg,n=6) at thermoneutrality for 28 weeks. Western blot was performed with antibody recognizing both human and mouse Cidea. mCidea arrow indicates expected position of mCidea. (c) Expression levels of adiponectin in eWAT and iWAT of wild-type (white bars) and transgenic (black bars) mice that have been on chow (wt,n=9; tg,n=5) or high-fat diet (wt,n=7; tg,n=6) at thermoneutrality for 28 weeks. (d–e) Representative western blot (d) and protein levels (e) of adiponectin in the serum of wild-type (white bars) and transgenic mice (black bars) that have been on chow (wt,n=6; tg,n=5) or high-fat diet (wt,n=6; tg,n=6) at thermoneutrality for 28 weeks. Values are means±s.e.m. *Significant difference between genotypes; *P<0.05; **P<0.01 by Student’st-test.#Significant difference between diets;#P<0.05;###P<0.001 by Student’st-test. The significance of diet effects on adiponectin expression levels in iWAT was not calculated because the expression of TATA-binding protein (TBP) in iWAT was affected by the diets (Supplementary Fig. 7a). Figure 5: Cidea permits perilipin retention in eWAT. ( a – b ) Representative western blots ( a ) and protein levels ( b ) of hCidea, perilipin 1, Akt and FABP4 in eWAT of wild-type (white bars) and transgenic mice (black bars) that have been on chow (wt, n =9; tg, n =5) or high-fat diet (wt, n =7; tg, n =6) at thermoneutrality for 28 weeks. Western blot was performed with antibody recognizing both human and mouse Cidea. mCidea arrow indicates expected position of mCidea. ( c ) Expression levels of adiponectin in eWAT and iWAT of wild-type (white bars) and transgenic (black bars) mice that have been on chow (wt, n =9; tg, n =5) or high-fat diet (wt, n =7; tg, n =6) at thermoneutrality for 28 weeks. ( d – e ) Representative western blot ( d ) and protein levels ( e ) of adiponectin in the serum of wild-type (white bars) and transgenic mice (black bars) that have been on chow (wt, n =6; tg, n =5) or high-fat diet (wt, n =6; tg, n =6) at thermoneutrality for 28 weeks. Values are means±s.e.m. *Significant difference between genotypes; * P <0.05; ** P <0.01 by Student’s t -test. # Significant difference between diets; # P <0.05; ### P <0.001 by Student’s t -test. The significance of diet effects on adiponectin expression levels in iWAT was not calculated because the expression of TATA-binding protein (TBP) in iWAT was affected by the diets ( Supplementary Fig. 7a ). Full size image White adipose tissue secretes a large set of endocrine and paracrine factors commonly referred to as adipokines [30] . The expression of adiponectin, an adipose tissue-specific adipokine with beneficial metabolic effects [30] , was almost abolished in eWAT of wild-type mice on high-fat diet ( Fig. 5c , top panel). However, in the transgenic mice, adiponectin mRNA levels were notably higher. Adiponectin mRNA levels were also significantly higher in iWAT of transgenic mice on either of diets ( Fig. 5c , bottom panel). Transgenic mice also had markedly higher circulating levels of adiponectin ( Fig. 5d,e ), highlighting the ability of Cidea to exert a constitutive stimulatory effect on adiponectin production and release. The effect was selective for adiponectin, as the expression levels of other adipokine genes ( Supplementary Figs 12a and 13a ) and adipose-selective genes ( Supplementary Figs 12b and 13b ) were not different between wild-type and transgenic mice on high-fat diet. In mice, the appearance of brite adipocytes in white fat depots (for example, during cold exposure) is accompanied by induction of Cidea expression [7] . Here we examined whether Cidea, merely by being present in white fat, would lead to its browning. Therefore, we measured expression levels of brown fat-specific/enriched genes (UCP1, DIO2 and PGC-1α) in eWAT and iWAT of wild-type and transgenic mice. Except for expression of PGC-1α in iWAT, the expression levels of brown fat-specific/enriched genes were below detection limit of quantitative PCR. Even the PGC-1α mRNA levels in iWAT were not affected by the presence of Cidea ( Supplementary Fig. 13b ). This is a clear demonstration that the white adipocytes that express Cidea under humanized conditions retain their ‘white’ identity. Thus, the presence of Cidea resulted in a qualitative difference between the wild-type and the transgenic visceral adipocytes, determining the health of the fat depot. Cidea does not inhibit fat mobilization It has been suggested that Cidea may regulate lipid storage by controlling lipolysis [31] , [32] . In in vitro systems, depletion of Cidea resulted in increased lipolysis [3] , [6] , whereas overexpression of Cidea led to reduced lipolysis and stimulated triglyceride storage [31] . However, it has not been investigated whether Cidea is involved in control of lipolysis in vivo . To determine whether impaired fat mobilization (lipolysis) may contribute to increased lipid storage in adipose tissue of transgenic mice, we placed wild-type and transgenic mice in metabolic chambers and monitored oxidative substrate preference during a 15-h fasting period. During prolonged fasting, triglyceride lipolysis and fatty acid oxidation are fully coupled. As demonstrated in Fig. 6a , both wild-type and transgenic mice experienced a similar dramatic decrease in respiratory exchange ratio (RER) in response to fasting; with increasing fasting time, the RER in both wild-type and transgenic mice decreased to ∼ 0.7 (the value for lipid oxidation), indicating a fully competent metabolic substrate switch to fatty acids oxidation. Furthermore, in response to injection of a β3-adrenergic agonist, similar increase in plasma free fatty acid and glycerol levels was observed in mice of two genotypes on chow diet ( Fig. 6b ); the RER in both wild-type and transgenic mice immediately dropped to 0.7 ( Fig. 6c ). In contrast, mouse models with defective lipolysis (adipose tissue triglyceride lipase (ATGL)-knockout mice [33] and mice with adipose overexpression of the lipolytic inhibitor G0/G1 switch gene 2 (ref. 34 )) are reported to be unable to mobilize and oxidize fat during fasting. Thus, the ability of aP2-hCidea mice to mobilize and oxidize fat demonstrates that Cidea does not inhibit lipolysis in vivo . 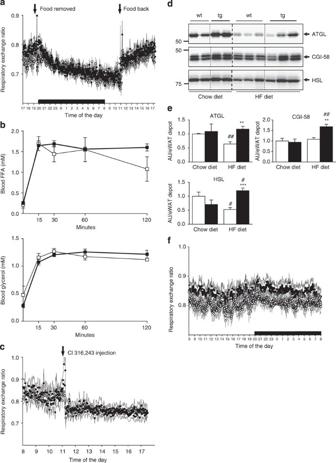Figure 6: Cidea does not inhibit fat mobilization. (a) Respiratory exchange ratio of wild-type (open symbols,n=6) and transgenic mice (filled symbols,n=7) living on high-fat diet at thermoneutrality for 5–6 months was analysed with indirect calorimetry at 30 °C as described in Methods. Food was removed at 2000 hours and given back the next day at 1100 hours (as indicated). Thin lines indicate s.e.m. (b) Lipolytic response of wild-type (open symbols,n=3) and transgenic mice (filled symbols,n=4) to CL316,243 injection (1 mg per kg body weight, i.p). Mice were living at thermoneutrality (on chow diet) for 2 months. Blood free fatty acids (FFA; top panel) and glycerol levels (lower panel) following CL316,243 injection. (c) Respiratory exchange ratio (RER) of wild-type (open symbols,n=5) and transgenic female mice (filled symbols,n=5) living at thermoneutrality on chow diet analysed with indirect calorimetry at 30 °C as described in Methods. Thin lines indicate s.e.m. The arrow indicates i.p. injection of Cl 316,243 at a dose of 1 mg kg−1body weight. (d–e) Representative western blots (d) and protein levels (e) of ATGL, CGI-58 and HSL in eWAT of wild-type (white bars) and transgenic mice (black bars) that have been on chow (wt,n=4–9; tg,n=5) or high-fat diet (wt,n=7; tg,n=6) at thermoneutrality for 28 weeks. Values are means±s.e.m. *Significant difference between genotypes; **P<0.01; ***P<0.001 by Student’st-test.#Significant difference between diets;#P<0.05;##P<0.01 by Student’st-test. (f) Respiratory exchange ratio of wild-type (open symbols,n=11) and transgenic mice (filled symbols,n=11) living on high-fat diet at thermoneutrality for 6 months was analysed with indirect calorimetry at 30 °C as described in Experimental Procedures. Thin lines indicate s.e.m. Figure 6: Cidea does not inhibit fat mobilization. ( a ) Respiratory exchange ratio of wild-type (open symbols, n =6) and transgenic mice (filled symbols, n =7) living on high-fat diet at thermoneutrality for 5–6 months was analysed with indirect calorimetry at 30 °C as described in Methods. Food was removed at 2000 hours and given back the next day at 1100 hours (as indicated). Thin lines indicate s.e.m. ( b ) Lipolytic response of wild-type (open symbols, n =3) and transgenic mice (filled symbols, n =4) to CL316,243 injection (1 mg per kg body weight, i.p). Mice were living at thermoneutrality (on chow diet) for 2 months. Blood free fatty acids (FFA; top panel) and glycerol levels (lower panel) following CL316,243 injection. ( c ) Respiratory exchange ratio (RER) of wild-type (open symbols, n =5) and transgenic female mice (filled symbols, n =5) living at thermoneutrality on chow diet analysed with indirect calorimetry at 30 °C as described in Methods. Thin lines indicate s.e.m. The arrow indicates i.p. injection of Cl 316,243 at a dose of 1 mg kg −1 body weight. ( d – e ) Representative western blots ( d ) and protein levels ( e ) of ATGL, CGI-58 and HSL in eWAT of wild-type (white bars) and transgenic mice (black bars) that have been on chow (wt, n =4–9; tg, n =5) or high-fat diet (wt, n =7; tg, n =6) at thermoneutrality for 28 weeks. Values are means±s.e.m. *Significant difference between genotypes; ** P <0.01; *** P <0.001 by Student’s t -test. # Significant difference between diets; # P <0.05; ## P <0.01 by Student’s t -test. ( f ) Respiratory exchange ratio of wild-type (open symbols, n =11) and transgenic mice (filled symbols, n =11) living on high-fat diet at thermoneutrality for 6 months was analysed with indirect calorimetry at 30 °C as described in Experimental Procedures. Thin lines indicate s.e.m. Full size image Molecular components of the lipolysis pathway are dysregulated by high-fat diet (ref. 35 and Fig. 5a,b ). However, as pointed out above, the loss of perilipin 1 in the eWAT of wild-type mice was fully prevented in the eWAT of transgenic mice ( Fig. 5a,b ). To examine whether other molecular components regulating lipolysis were affected by the presence of Cidea, we measured protein levels of ATGL, ATGL co-lipase CGI-58 and hormone-sensitive lipase (HSL). Protein levels of ATGL and HSL in eWAT of wild-type mice were significantly decreased as a consequence of prolonged high-fat diet ( Fig. 6d,e ). Remarkably, the lipase levels were fully retained and CGI-58 levels were even increased in the eWAT of transgenic mice. The lipases levels in iWAT were not significantly affected by the presence of Cidea ( Supplementary Fig. 14 ). To examine whether the expression of Cidea in adipose tissues affected metabolic substrate preference under non-extreme metabolic demands (that is, during ad libitum feeding), high-fat diet-fed wild-type and aP2-hCidea mice were subjected to a metabolic chamber study and RER values were monitored during a 24-h period in the presence of ad libitum food. When compared with wild-type mice, aP2-hCidea mice exhibited markedly higher RER values ( Fig. 6f ). Thus, transgenic mice preferentially utilized carbohydrates as a metabolic substrate, which implies that lipids were more readily stored than oxidized. Amelioration of insulin sensitivity in aP2-hCidea mice Preferential utilization of carbohydrates as a metabolic substrate, as well as increased circulating levels of adiponectin and retention of Akt in eWAT, suggests improved glucose metabolism in the transgenic mice. Therefore, we examined glucose homeostasis in these mice. Diet-induced obesity is frequently associated with impaired glucose tolerance and type 2 diabetes [36] , [37] . However, aP2-hCidea mice, despite being significantly more obese, had blood-glucose profiles similar to the wild-type mice, as revealed by an i.p. glucose tolerance test ( Fig. 7a ). As seen, glucose disposal, as estimated by the glucose disposal rate constant ( K G ), was markedly higher in transgenic (0.52±0.06%/min) than in wild-type mice (0.32±0.08% per min; P <0.08 by Student’s t -test; Fig. 7b ). Similarly, an insulin tolerance test demonstrated improved insulin sensitivity ( Fig. 7c and Supplementary Fig. 15b ), as well as significantly increased insulin-induced glucose disposal in transgenic mice (the glucose disposal rate constant was 1.35±0.34% per min in wild-type versus 2.05±0.34% per min in transgenic mice, P <0.05 by Student’s t -test; Fig. 7d ). Furthermore, an oral glucose tolerance test revealed significantly improved blood-glucose profiles in aP2-hCidea mice ( Fig. 7e ), with increased glucose disposal rate constant (0.28±0.02% per min in wild-type versus 0.39±0.05% per min in transgenic mice, P <0.05 by Student’s t -test; Fig. 7f ). Insulin levels, both basal and glucose-induced, were lower in transgenic mice ( Fig. 7g,h ), again indicating improvement of insulin sensitivity in transgenic mice. The values of the homeostasis model assessment of insulin resistance, a surrogate marker of insulin resistance [38] , were also consistent with improved glucose metabolism in aP2-hCidea mice ( Fig. 7i ). Thus, despite being significantly more obese, aP2-hCidea mice displayed higher insulin sensitivity. 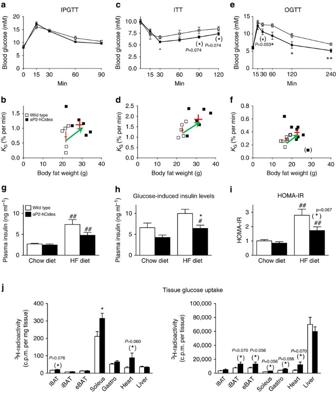Figure 7: Amelioration of insulin sensitivity in aP2-hCidea mice. (a,b) Intraperitoneal glucose tolerance test. (a) Blood glucose levels during an intraperitoneal glucose tolerance test in fasted wild-type and transgenic mice fed with high-fat diet for 25 weeks. (b) Correlation between body fat weight and glucose disposal rate constant (KG), based ona. (c,d) Insulin tolerance test. (c) Blood glucose levels during an intraperitoneal insulin tolerance test. A single dose of insulin was given to fasted wild-type (n=5) and transgenic mice (n=6) fed with high-fat diet for 33 weeks. (d) Correlation between body fat weight and insulin-induced glucose disposal rate constant (KG), based onc. (e,f) Oral glucose tolerance test. (e) Blood glucose levels during an oral glucose tolerance test in fasted wild-type (n=8) and transgenic mice (n=8) fed with high-fat diet for 25 weeks. (f) Correlation between body fat weight and glucose disposal rate constant (KG), based one. (g–i) Fasting and glucose-induced insulin levels in mice examined inaand inSupplementary Fig. 15a(one outlier wild-type mouse on chow diet and one outlier transgenic mouse on high-fat diet were excluded from the calculations). Serum was collected after (g) 6 h of fasting and (h) 15 min after injection of glucose. (i) Homeostasis model assessment of insulin (HOMA-IR). (j) Glucose uptake in various tissues of wild-type (n=8) and transgenic mice (n=8) fed with high-fat diet at thermoneutrality for∼25 weeks (the mice examined ine). A single gavage of glucose was given to fasted mice. Glucose uptake was determined 240 min after gavage (as described in Experimental Procedures). Values shown ina,c,eandg–jare means±s.e.m. Crosses shown inb,d,frepresent mean values±s.e.m. Arrows denote the direction ofKGchanges induced by the expression of Cidea.*Significant difference between genotypes; *P<0.05 by Student’st-test.#Significant difference between diets;#P<0.05;##P<0.01 by Student’st-test. Figure 7: Amelioration of insulin sensitivity in aP2-hCidea mice. ( a , b ) Intraperitoneal glucose tolerance test. ( a ) Blood glucose levels during an intraperitoneal glucose tolerance test in fasted wild-type and transgenic mice fed with high-fat diet for 25 weeks. ( b ) Correlation between body fat weight and glucose disposal rate constant ( K G ), based on a . ( c , d ) Insulin tolerance test. ( c ) Blood glucose levels during an intraperitoneal insulin tolerance test. A single dose of insulin was given to fasted wild-type ( n =5) and transgenic mice ( n =6) fed with high-fat diet for 33 weeks. ( d ) Correlation between body fat weight and insulin-induced glucose disposal rate constant ( K G ), based on c . ( e , f ) Oral glucose tolerance test. ( e ) Blood glucose levels during an oral glucose tolerance test in fasted wild-type ( n =8) and transgenic mice ( n =8) fed with high-fat diet for 25 weeks. ( f ) Correlation between body fat weight and glucose disposal rate constant ( K G ), based on e . ( g – i ) Fasting and glucose-induced insulin levels in mice examined in a and in Supplementary Fig. 15a (one outlier wild-type mouse on chow diet and one outlier transgenic mouse on high-fat diet were excluded from the calculations). Serum was collected after ( g ) 6 h of fasting and ( h ) 15 min after injection of glucose. ( i ) Homeostasis model assessment of insulin (HOMA-IR). ( j ) Glucose uptake in various tissues of wild-type ( n =8) and transgenic mice ( n =8) fed with high-fat diet at thermoneutrality for ∼ 25 weeks (the mice examined in e ). A single gavage of glucose was given to fasted mice. Glucose uptake was determined 240 min after gavage (as described in Experimental Procedures). Values shown in a , c , e and g – j are means±s.e.m. Crosses shown in b , d , f represent mean values±s.e.m. Arrows denote the direction of K G changes induced by the expression of Cidea. *Significant difference between genotypes; * P <0.05 by Student’s t -test. # Significant difference between diets; # P <0.05; ## P <0.01 by Student’s t -test. Full size image To determine which peripheral tissues were responsible for the improved insulin action in transgenic animals, we measured glucose uptake in peripheral organs after an oral glucose tolerance test. Glucose uptake measured in this experimental setup reflects physiological postprandial glucose uptake driven by hyperglycemia-induced hyperinsulinemia ( Supplementary Fig. 15c ). As demonstrated in Fig. 7j , glucose uptake was increased in almost all insulin-sensitive tissues of the transgenic animals, particularly in oxidative skeletal muscle (soleus) and heart. To assess liver insulin sensitivity, we performed alanine tolerance test (principally as described in ref. 39 ). Alanine, in contrast to glycerol or pyruvate, is an exclusive hepatic substrate. Importantly, both wild-type and transgenic mice significantly increased plasma glucose levels in response to alanine injection after 16 h of fasting ( Supplementary Fig. 15d ), a time when glycogen stores were exhausted and liver gluconeogenesis enhanced. Although glucose levels were consistently lower in transgenic mice, the overall response to alanine injection was similar to wild-type mice, demonstrating that the hepatic glucose output was not affected by the presence of Cidea in white fat. Thus, unaltered liver gluconeogenic response as well as unaltered liver glucose uptake ( Fig. 7j ) demonstrate that the liver insulin sensitivity was not affected by the presence of Cidea in white fat. The widely accepted view that considers obesity as the major factor leading to insulin resistance contrasts with our observations. Our data clearly indicate that it is not the obesity per se , but rather the (in)ability of adipose tissue to expand, together with its physiological healthiness, that play significant roles in determining the propensity to develop metabolic complications, being fully in agreement with the adipose tissue expandability hypothesis [40] . Notably, the ameliorated insulin sensitivity observed in aP2-hCidea mice cannot be explained by a difference in the total number of macrophages in eWAT or by an altered ratio of the M1/M2 macrophages towards a less inflammatory state (see above). As the major effects of Cidea expression were observed in the eWAT of the transgenic mice, we propose that this fat depot has significant impact on systemic insulin sensitivity. In other mouse models of healthy obesity (in mice overexpressing adiponectin [41] or mitoNEET [42] in adipose tissue), as well as in mice treated with thiazolidinediones (TZDs) [41] , the improvements in insulin sensitivity were mainly caused by an expansion of subcutaneous iWAT. However, we show that the visceral (eWAT) fat of transgenic mice, when protected against the detrimental effects that a high-fat diet exerts on its functionality, also plays a beneficial role in systemic glucose metabolism. It may be noted that in our mouse model, the remarkable systemic effects caused by Cidea expression in adipose tissues were displayed on a normal C57Bl/6 background. In contrast, the effects of adiponectin [41] , mitoNEET [42] or the effects of adipose-specific ablation of PPARγ2 (ref. 43 ), were prominent only in the context of an ob/ob background. We have developed a mouse model that has allowed us to establish a role for Cidea in human energy metabolism. We demonstrate that mice expressing human Cidea in white fat display a metabolically healthy obesity. Mechanistically, the data can be visualized in the model summarized in Fig. 8 . In the wild-type mice, the (epididymal) fat cells are coping well with the normal input of fatty acids. The lipid stores in the cells are covered with perilipin, and the adipocytes are therefore functionally intact. When these mice are exposed to an excess of fatty acids, such as when the mice are offered a high-fat diet, adipocyte hypertrophy [13] and preadipocyte hyperplasia [15] , [16] are initiated. However, prolonged exposure to high-fat diet invokes hypertrophy-associated death of epididymal adipocytes [13] and shrinkage of the entire eWAT ( Fig. 8 , top-right mouse); the tissue is invaded with macrophages that both clean up dead adipocytes and release proinflammatory cytokines [13] , [20] , [21] . Consequently, the remaining adipocytes are severely damaged (as demonstrated by the absence of perilipin 1), are non-functional (incompetent to produce adiponectin) and insulin-resistant (Akt deficient), which contributes to the development of systemic insulin resistance and poor health. 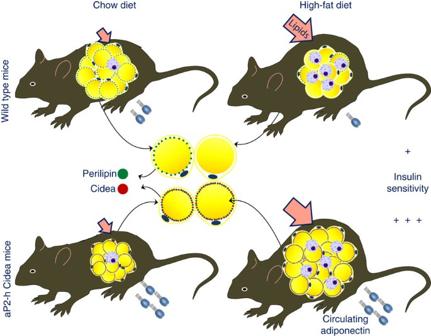Figure 8: Proposed mechanism of Cidea function. As a response to high-fat diet, the visceral (epididymal) fat depot (represented by the yellow adipocytes) changes its size in qualitatively different ways: in wild-type mice, the tissue becomes smaller while in transgenic mice it becomes larger. Note the same number of macrophages (blue cells) per total fat depot in both strains. Under humanized conditions, wild-type adipocytes lose virtually all perilipin 1 (green dots), Akt (not shown) and adiponectin (indicated outside the mouse for clarity). Transgenic adipocytes (that express Cidea (red dots)) retain perilipin 1, Akt and adiponectin expression/secretion. Transgenic mice, as a consequence of these retained molecular characteristics and preserved expandability of visceral adipose depots, exhibit ameliorated insulin sensitivity. Figure 8: Proposed mechanism of Cidea function. As a response to high-fat diet, the visceral (epididymal) fat depot (represented by the yellow adipocytes) changes its size in qualitatively different ways: in wild-type mice, the tissue becomes smaller while in transgenic mice it becomes larger. Note the same number of macrophages (blue cells) per total fat depot in both strains. Under humanized conditions, wild-type adipocytes lose virtually all perilipin 1 (green dots), Akt (not shown) and adiponectin (indicated outside the mouse for clarity). Transgenic adipocytes (that express Cidea (red dots)) retain perilipin 1, Akt and adiponectin expression/secretion. Transgenic mice, as a consequence of these retained molecular characteristics and preserved expandability of visceral adipose depots, exhibit ameliorated insulin sensitivity. Full size image The presence of Cidea in the adipocytes dramatically alters the prognosis. In the non-challenged mice (on a chow diet), Cidea has limited effect on adipocyte function. However, when the transgenic mice are exposed to the prolonged lipid challenge, the presence of Cidea in the epididymal adipocytes enables their survival and protects their functionality ( Fig. 8 , bottom-right mouse). The presence of Cidea allows protection of perilipin 1 protein, the adipocytes are subsequently able to enlarge (competent in accumulating surplus triglycerides), functional (competent in producing adiponectin) and insulin-sensitive (Akt replete), constituting a significantly expanded eWAT. Thus, both the plasticity and the expandability of eWAT are rescued by the presence of Cidea. Function of Cidea in enlargement of lipid droplets and enhancement of adipose tissue lipid storage capacity is substantiated by the phenotype of eWAT in Cidea/Fsp27 double-deficient mice [44] . In comparison to eWAT of only Fsp27-deficient mice, which (compensatorily) expresses Cidea, eWAT of double-deficient mice had significantly decreased lipid storage capacity and had accumulated numerous very small lipid droplets. By being efficient in extracting fatty acids from the circulation, Cidea-containing adipocytes protect the rest of the body from both excessive fatty acid exposure and ectopic triglyceride accumulation (the liver accumulates less fat, and hepatosteatosis is thus reduced). This is in line with the altered metabolic substrate utilization in the transgenic mice: preferential utilization of carbohydrates and storage of lipids. However, during instances of increased metabolic demand (such as fasting or β3-adrenergic stimulation), Cidea does not inhibit mobilization of the fatty acids from triglyceride stores and therefore allows the important metabolic switch from carbohydrates to fatty acids. The increased circulating levels of adiponectin also contribute to the preferential storage of triglycerides in adipose tissue [41] and improve metabolic flexibility and insulin sensitivity [40] , [45] . This mechanistic scenario harmonizes well with the observations in humans where the presence of Cidea in white adipose tissue is associated with a healthier type of obesity [1] , [3] , [5] . Also in humans, visceral adipose depots are particularly sensitive to nutrient overload, determining the propensity to develop the metabolic complications of obesity [46] . Insulin resistance in obese individuals is suggested to occur as a result of their inability to respond to the need to store excess energy (triacylglycerol) by increasing the production of fully differentiated, mature adipose cells [47] . However, obese subjects who express high levels of Cidea in visceral depots are protected from these metabolic complications [1] . Whereas these data in humans are only correlative, we demonstrate here that it is the presence of Cidea in itself that is causative, that is, confers upon the white adipose cells the ability to withstand the pressure of augmented fatty acid load and thus to remain healthy, leading to a healthier obese phenotype both in mice and humans. Generation of transgenic mice Adipose-specific human Cidea transgenic mice were generated by subcloning human Cidea into a plasmid containing the 5.4-kb aP2 promoter. A plasmid containing the aP2 gene-promoter in pBluescript II SK was created by Dr B. M. Spiegelman [48] and purchased from Addgene. A 5.6-kb Sal I- Not I fragment of the aP2-promoter was subcloned in a pCI vector (Promega)—designated as aP2-pCI. The human Cidea (hCidea) full open reading frame cDNA was originally cloned in a pcDNA vector (Invitrogen) [49] . The full open reading frame of hCidea was reamplified by PCR using primers containing Not I-restriction site overhangs. The PCR product was cut with Not I and subcloned into the NotI site of aP2-pCI—designated as aP2-hCidea-pCI. Plasmids with correct orientation were selected and sent for sequencing (Eurofins MWG/Operon, Germany). Then, plasmids with a confirmed hCidea sequence were amplified and linearized with ClaI. Finally, after linearization, a 6.6-kb-long construct, containing the aP2-promoter fused to the hCidea cDNA, followed by a 3′- polyadenylation signal (from the pCI vector), was sent to the Karolinska Center for Transgenic Technologies, where pronuclear injections onto a C57Bl/6 background were performed. Founder mice were analysed by PCR for the presence of the transgenic insert in the genomic DNA (specific primers used were 5′-CCAGGGAGAACCAAAGTTGA-3′ and 5′-GAAACTGTCCCGTCACCTG-3′). Successful germ-line transmission was confirmed in four positively identified founders, hereafter named as the aP2-hCidea mice. However, we chose to investigate the line in which the human Cidea was expressed in both brown and white adipose tissue at levels similar to the levels of the native mouse Cidea in brown fat ( Fig. 1 ). In two transgenic lines (lines 76 and 85), human Cidea was expressed at levels lower than the levels of mouse Cidea in brown fat; in the fourth transgenic line (line 67), the levels of human Cidea were high in brown fat and very low in white fat ( Supplementary Fig. 1 ). The aP2-hCidea transgenic mice were maintained by crossing the heterozygous transgenic mice to wild-type C57Bl/6 mice. Metabolic studies All experiments were approved by the Animal Ethics Committee of the North Stockholm region. Before the start of the experiment, all mice were housed at 22–24 °C with a 12:12-h light–dark cycle, with free access to food (R70, Lactamin) and water. At the start of the experiment, 12-week-old male mice were single caged and transferred to 30 °C (thermoneutrality). The control-diet mice had access only to chow (R70, Lactamin) and the high-fat-fed mice had access only to high-fat diet (45% calories from fat, Research Diets D12451). All groups had free access to water and food (unless otherwise stated) and 12:12-h light–dark cycle regime. The mice were kept at thermoneutrality for at least 25 weeks. Body weight and body composition were measured when indicated. The body composition of the mice was measured with a magnetic resonance imaging technique (EchoMRI-700/100 Body Composition Analyzer, Echo Medical Systems). Food intake was measured between weeks 8 and 10; food was weighed when supplied and remaining food (including spillage and so on) was subtracted. The energy content of the food ingested was calculated based on data from the manufacturers of the food. Indirect calorimetry For indirect calorimetry, the INCA System was used (Somedic). Before the start of an experiment, the equipment was calibrated with reference gases (15 and 25% O 2 in N 2 ). The airflow was 1 l min −1 . Energy metabolism was examined during week 12 and weeks 22–25 at thermoneutrality. To obtain daily energy expenditure (EE), the mice were placed during late afternoon (that is, at the end of their inactive phase) in the 4-l metabolic chambers at 30 °C in their home cages. Every 2nd minute for ∼ 38 h, O 2 consumption and CO 2 production were recorded and the RER value was calculated (RER=volume CO 2 /volume O 2 ). Theoretical RER value for the chow diet is 0.95 and for the high-fat diet is 0.84. EE, adjusted for lean weight, was calculated using the Weir equation (EE (mW)=(16.3 × volume O 2 (ml)+4.57 × volume CO 2 (ml)) × 16.67 (ref. 50 ). It was calculated for a period of 24 h, starting at 0800 hours ( ∼ 14 h after the mice have been placed in the chambers). To obtain RER values during fasting and as a response to β3-agonist injection, the experiments were performed as indicated on corresponding figures ( Fig. 6a,c , respectively). Intraperitoneal glucose tolerance test (GTT) The food was removed 6–8 h before the initiation of a GTT. GTT was performed at the ambient temperature of 30 °C. Blood was collected from a small incision in the tip of the tail (time 0) and then 15, 30, 60 and 90 min after an i.p. injection of glucose (1 g kg −1 lean body weight). Blood glucose levels were measured with a blood glucometer (Accu-Check Aviva, Roche). The glucose disposal rate was quantified as the glucose disposal rate constant ( K G ), the reduction in circulating glucose between minutes 15 and 60 after i.p. administration, after logarithmic (ln) transformation of the individual blood glucose values, and expressed as percent disposal of glucose per minute [37] . Blood samples for insulin measurement were collected with capillary tubes (Microvette CB300, Sarstedt) at times 0 and 15 min after glucose challenge. The serum insulin levels were determined using an Ultrasensitive Mouse Insulin ELISA kit (Chrystal Chem Inc.). Homeostasis model assessment of insulin resistance was calculated as (fasting glucose level × fasting insulin level)/22.4 (ref. 38 ). Oral GTT and glucose uptake The food was removed 14–16 h before the initiation of a GTT. GTT was performed at the ambient temperature of 30 °C. Blood was collected from a small incision in the tip of the tail (time 0) and then 15, 30, 60, 120 and 240 min after an gavage of glucose (1.4 g glucose per kg lean body weight traced with 12.8 MBq 3 H-Deoxyglucose per kg lean body weight) immediately followed by another gavage of olive oil (4 ml olive oil per kg lean body weight). Blood glucose levels were measured with a blood glucometer (Accu-Check Aviva, Roche). The glucose disposal rate was quantified as the glucose disposal rate constant ( K G ), the reduction in circulating glucose between minutes 15 and 240 after gavage, after logarithmic (ln) transformation of the individual blood glucose values, and expressed as percent disposal of glucose per minute [37] . The animals were killed 240 min after gavage by CO 2 anaesthesia and immediately perfused with PBS. Multiple tissues (those presented on Fig. 7j ) have been dissected, weighted and lysed in 10 volumes of 0.5 M NaOH. Radioactivity was measured by liquid scintillation counting (200 μl of lysate in 4 ml of Emulsifier-Safe, Perkin Elmer). Insulin tolerance test (ITT) The food was removed 4–6 h before the initiation of an ITT. The ITT was performed at the ambient temperature of 30 °C. Blood was collected from a small incision in the tip of the tail (time 0) and then 15, 30, 60, 90 and 120 min after an i.p. injection of insulin (0.75 U kg −1 body weight; Actrapid Penfill, Novo Nordisk). Blood glucose levels were measured with a blood glucometer (Accu-Check Aviva, Roche). The glucose disposal rate was quantified as the glucose disposal rate constant ( K G ), the reduction in circulating glucose between minutes 0 and 30 after i.p. administration, after logarithmic (ln) transformation of the individual blood glucose values, and expressed as percent disposal of glucose per minute [37] . Alanine tolerance test (ATT) The food was removed 14–16 h before the initiation of an ATT. The ATT was performed at the ambient temperature of 30 °C. Blood was collected from a small incision in the tip of the tail (time 0) and then 15, 30, 60, 90 and 120 min after an i.p. injection of alanine (2.8 g per kg lean body weight). Blood glucose levels were measured with a blood glucometer (Accu-Check Aviva, Roche). Free fatty acids measurement Serum free fatty acid levels were determined with enzymatic colorimetric assay (Half-micro test, Roche). Glycerol and triglycerides measurement Serum glycerol and triglyceride levels were measured sequentially using Serum Triglyceride Determination Kit (Sigma-Aldrich). Sampling of tissues The animals were killed by CO 2 anaesthesia. The blood was collected by cardiac puncture; serum was obtained by centrifuging coagulated blood at 10,000 g for 5 min. Interscapular brown adipose tissue, inguinal white adipose tissue and epididymal white adipose tissue were quantitatively dissected. The left and the right lobes/depots of adipose tissues were placed in separate tubes and were either directly frozen in liquid nitrogen and stored at −80 °C or fixed in formaldehyde solution for histological analysis. Quantitative real-time PCR Total RNA was extracted from frozen adipose tissue (left pad) with TRI Reagent (Sigma-Aldrich) according to the manufacturer’s protocol, and RNA concentrations were measured on a Nanodrop nd-1000 spectrophotometer (Thermo-Scientific). To synthesize cDNA, 500 ng of RNA were reverse-transcribed with a High Capacity cDNA kit (Applied Biosystems) in a total volume of 20 μl. Primers ( Supplementary Table 3 ) were pre-mixed with SYBR Green JumpStart Taq ReadyMix (Sigma-Aldrich), and aliquots of 11 μl were applied to 96-well Multiplate PCR Plates (Bio-Rad). cDNA was diluted 1:10, and aliquots of 2 μl were added in triplicates. Thermal cycling conditions were: 2 min at 50 °C, 10 min at 95 °C and 40 cycles of 15 s at 95 °C and 1 min at 65 °C on a CFX Connect Real-Time System (Bio-Rad). The Δ C t method was used to calculate relative changes in mRNA abundance. The threshold cycle ( C t ) for TATA-binding protein was subtracted from the C t for the target gene to adjust for variations in the cDNA synthesis. Western blot The right pad of the epididymal white adipose tissue was homogenized in modified RIPA buffer (50 mM Tris-HCl, pH 7.4, 1% Triton X-100, 150 mM NaCl, 1 mM EDTA) with freshly added 1 mM Na 3 VO 4 , 10 mM NaF and protease inhibitor cocktail (Complete-Mini, Roche). The homogenates, after freezing (in liquid nitrogen) and defrosting—in order to fully lyse adipose cells—were centrifuged at 14,000 g for 15 min. The top fat layer was discarded and the lysate (infranatant) carefully aspirated using a 1-ml syringe and 27-G needle. The concentration of proteins in the lysate was determined using the method of Lowry. An equal volume of reducing sample buffer (62.5 mM Tris·HCl, pH 6.8, 2% (wt/vol) SDS, 10% (vol/vol) glycerol, 100 mM dithiothreitol, and 0.1% (wt/vol) bromphenol blue) was added to each sample. To determine circulating adiponectin levels, 9 volumes of reducing sample buffer (27 μl) were added to 1 volume of serum (3 μl). Proteins were separated by SDS–PAGE in ordinary 12% polyacrylamide gel (acrylamide/bis-acrylamide=37.5/1), except for determination of F4/80 when the proteins were separated in highly porous 12% polyacrylamide gel (acrylamide/bis-acrylamide=175/1) with high-resolution capacity under non-reducing conditions. Proteins were transferred to polyvinylidene difluoride membranes (GE Healthcare Life Sciences) in 48 mM Tris·HCl, 39 mM glycine, 0.037 (wt/vol) SDS and 15% (vol/vol) methanol using a semi-dry electrophoretic transfer cell (Bio-Rad Trans-Blot SD; Bio-Rad) at 1.2 mA cm −2 for 90 min. After transfer, the membrane was stained with Ponceau S for examination of equal loading of proteins. After being washed, the membrane was blocked in 5% milk in Tris-buffered saline-Tween for 1 h at room temperature and probed with the indicated antibodies overnight at 4 °C. The immunoblot was visualized with appropriate horseradish peroxidase-conjugated secondary antibodies and enhanced chemiluminescence (ECL kit, GE Healthcare Life Sciences) in a charge-coupled device camera (Fuji Film). Unedited blots are shown in Supplementary Fig. 16 . Antibodies used were as follows: Cidea antibody specific for human Cidea (Sigma-Aldrich, C7987), diluted 1:1,000; Cidea antibody recognizing both mouse and human Cidea (Santa Cruz Laboratories, sc-8730-R), diluted 1:1,000; perilipin antibody (Cell Signaling, 9349), diluted 1:2,000; pan-Akt antibody (Cell Signaling, 2929), diluted 1:2,000; FABP4 antibody (Cell Signaling, 3544), diluted 1:2,000; MAC-2 antibody (Santa Cruz Laboratories, sc-23938), diluted 1:5,000; F4/80 antibody (Molecular Probes, MF48000), diluted 1:300; adiponectin antibody (Cell Signaling, 2789), diluted 1:1,000; ATGL antibody (Cell Signaling, 2439), diluted 1:1,000; HSL antibody (Cell Signaling, 2439), diluted 1:1,000 and CGI-58 antibody (Abcam, ab183739), diluted 1:1,000. In vitro transcription/translation Plasmid (pSV Sport) containing the full-length human Cidea cDNA sequence was used as template for in vitro transcription/translation in the TnT SP6 Quick coupled reticulocyte lysate (Promega), according to the manufacturer’s protocol. Briefly, a total of 1 μg of plasmid DNA was transcribed/translated in a 50-μl reaction sample incubated for 90 min at 30 °C. Two microlitres of reaction mix was separated by SDS–PAGE in ordinary 12% polyacrylamide gel, in parallel with tissue lysates. Histology The right lobe/pad of the interscapular brown adipose tissue, inguinal white adipose tissue, epididymal white adipose tissue and samples of liver were immersion-fixed in 4% alcoholic formaldehyde (4% formaldehyde in ethanol) for 24 h, then dehydrated and embedded in paraffin by a standard procedure [51] . Tissues were sectioned using standard microtome (Leica RM2255, Leica Microsystems). Sections, 5 μm thick, were mounted on SuperFrost Plus adhesion slides (VWR International bvba,), then deparaffinized, rehydrated and stained with haematoxylin and eosin or picrosirius red. Adipocyte diameters were measured on haematoxylin and eosin stained slides using Adiposoft software [52] . Determination of liver fat content Pieces of liver ( ∼ 200 mg) were placed in preweighed glass vials and weighed ((wet weight) as described in ref. 53 ). To each vial, 5 ml methanol:chloroform (1:2, vol/vol) were added, and the tissue was extracted at room temperature for 2 days. The extraction medium was then transferred to another preweighed vial (the lipid vial), and a further 2 ml of the same extraction medium were added to the original vial. Two days later, this extract was added to the previous extract in the lipid vial. The extraction medium in the lipid vial was evaporated, and the lipid weight was determined gravimetrically and expressed as percentage of wet tissue weight. How to cite this article : Abreu-Vieira, G. et al. Cidea improves the metabolic profile through expansion of adipose tissue. Nat. Commun. 6:7433 doi: 10.1038/ncomms8433 (2015).